Visualization of exciton transport in ordered and disordered molecular solids Transport of nanoscale energy in the form of excitons is at the core of photosynthesis and the operation of a wide range of nanostructured optoelectronic devices such as solar cells, light-emitting diodes and excitonic transistors. Of particular importance is the relationship between exciton transport and nanoscale disorder, the defining characteristic of molecular and nanostructured materials. Here we report a spatial, temporal and spectral visualization of exciton transport in molecular crystals and disordered thin films. Using tetracene as an archetype molecular crystal, the imaging reveals that exciton transport occurs by random walk diffusion, with a transition to subdiffusion as excitons become trapped. By controlling the morphology of the thin film, we show that this transition to subdiffusive transport occurs at earlier times as disorder is increased. Our findings demonstrate that the mechanism of exciton transport depends strongly on the nanoscale morphology, which has wide implications for the design of excitonic materials and devices. Energy transport in nanostructured thin films and crystals (such as those composed of molecules, polymers and colloidal quantum dots) occurs by the motion of tightly bound electron-hole pairs, known as excitons [1] . Exciton transport is at the core of photosynthesis [2] , [3] and it similarly governs the operation of a wide array of nanostructured optoelectronic devices including molecular, polymeric and colloidal-quantum-dot solar cells [4] , [5] , light-emitting diodes [6] and excitonic transistors [7] . For example, in molecular and polymeric solar cells, excitons are generated by absorption of sunlight, and must be moved efficiently to an interface where electron and hole are separated to produce charge buildup, leading to photovoltage and photocurrent. Likewise, the efficient transport of photogenerated excitons from the light-harvesting complex of a plant to the reaction centre is at the core of photosynthesis [2] . Understanding and manipulating the flow of excitons in such systems can enhance device performance [5] and can lead to development of next-generation excitonic technologies. The motion of excitons in molecular solids is thought to occur by transfer of the localized excitation to a neighbouring molecular site, resulting in random walk diffusion [8] , [9] . Two types of hopping mechanisms are possible: For excitons in the radiative spin singlet state (electronic spin of zero), hopping occurs by Förster energy transfer, a near-field dipole–dipole interaction, with interaction distance of the order of 5 nm [1] . Excitons that are in the triplet state (electronic spin of one) are spin-forbidden from emitting, and hence triplet exciton hopping is dominated by Dexter energy transfer. This energy transfer process is a simultaneous exchange of two electrons between nearest molecular neighbours, the rate of which depends on the spatial and energetic overlap of the two molecular wavefunctions. While band transport of excitons has been studied extensively [10] , [11] , [12] , [13] , mostly indirect methods have been utilized to measure exciton propagation in materials with localized excitons due to their shorter propagation lengths. These techniques include optoelectronic device modelling [14] , exciton quenching at a surface or an interface [4] , [6] , [15] , [16] , and exciton-density-dependent exciton–exciton annihilation [17] . Such approaches produce only an average ‘diffusion length’, L D , defined as the mean displacement of an exciton during its lifetime, but no direct evidence exists that exciton transport occurs by hopping-driven diffusion. A limited number of studies on molecular solids have used imaging of exciton photoluminescence [18] , [19] , however, these approaches relied on steady-state excitation, obscuring the temporal dynamics of exciton transport. Müller and Bardeen [20] used time-resolved microscopy to image transport, but did not detect energy migration in a molecular solid. Diffraction from exciton density gratings has been used to study dynamics of exciton transport [21] , but this approach requires high exciton densities to be created, which introduces challenges such as exciton–exciton interactions and material damage. Due to the lack of a general technique, the temporal dynamics of exciton transport in molecular solids and how it relates to the nanoscale disorder, the defining characteristic of molecular and nanostructured materials, remains elusive. Here, we report a spatial, temporal and spectral visualization of exciton transport in crystals and thin films of tetracene, a well-studied organic semiconductor in which triplet excitons are dominant [22] , [23] . We reveal that exciton transport occurs by random walk diffusion, with a transition to subdiffusion as excitons become trapped. By controlling the morphology of the thin film, we show that this transition to subdiffusive transport occurs at earlier times as disorder is increased. Our findings demonstrate that the mechanism of exciton transport depends strongly on the nanoscale morphology of molecular materials, which has wide implications for the design of excitonic materials and devices. Experimental setup Tetracene is an archetypal test bed for the study of exciton transport both because acenes have been studied as excitonic photovoltaic materials [24] and because tetracene film morphology and crystallinity can be tuned. Upon optical excitation of tetracene at λ =400 nm, singlet excitons are generated, and undergo rapid fission into two triplet excitons, each with slightly more than one half the energy of the singlet ( Fig. 1a,b ) [25] . Some of the photogenerated singlets decay radiatively, which is known as the prompt fluorescence process, with a lifetime of τ PF =262 ps ( Fig. 1c ). The triplet excitons undergo random hopping to the nearest neighbour molecular sites by Dexter energy transfer. When two diffusing triplets encounter each other, triplet fusion can occur to produce a singlet exciton. The subsequent radiative relaxation of the formed singlet exciton, known as delayed fluorescence ( τ DF =1.37 μs), can be optically detected and used as a direct probe of the triplet exciton density. 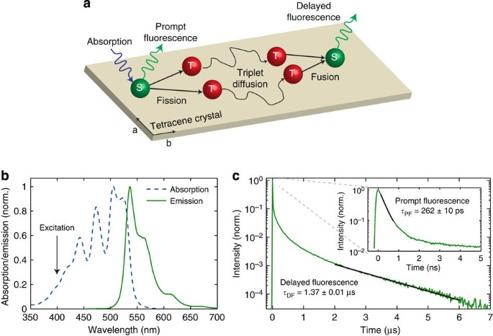Figure 1: Excitonic and optical properties of tetracene. (a) Excitonic processes in tetracene films and crystals that are relevant to this study. Upon absorption a singlet exciton is generated. Some singlets decay radiatively (prompt fluorescence) while a significant fraction decays into two triplet excitons, each with slightly more than half the energy of the singlet. Through diffusion two triplets can collide to again produce a singlet that can decay radiatively (delayed fluorescence). (b) Absorption spectrum of a tetracene thin film and steady-state emission spectrum of a tetracene single crystal. The transport measurements are done on films and crystals excited at a laser excitation wavelength ofλ=400 nm. (c) Time-resolved photoluminescence decay from a tetracene single crystal showing the regimes of prompt and delayed fluorescence. norm., normalized. Figure 1: Excitonic and optical properties of tetracene. ( a ) Excitonic processes in tetracene films and crystals that are relevant to this study. Upon absorption a singlet exciton is generated. Some singlets decay radiatively (prompt fluorescence) while a significant fraction decays into two triplet excitons, each with slightly more than half the energy of the singlet. Through diffusion two triplets can collide to again produce a singlet that can decay radiatively (delayed fluorescence). ( b ) Absorption spectrum of a tetracene thin film and steady-state emission spectrum of a tetracene single crystal. The transport measurements are done on films and crystals excited at a laser excitation wavelength of λ =400 nm. ( c ) Time-resolved photoluminescence decay from a tetracene single crystal showing the regimes of prompt and delayed fluorescence. norm., normalized. Full size image To measure triplet exciton transport in tetracene thin films and crystals, a λ =400 nm wavelength 100 fs pulsed laser excitation is focused to a near-diffraction-limited spot, generating an in-plane Gaussian distribution of singlet excitons within an absorption length 1/ α abs =1.3 μm of the surface, where α abs is the absorption coefficient ( Fig. 2a,b ). The delayed fluorescence resulting from triplet fusion is imaged with × 500 magnification onto a time-resolved single photon counting detector. The detector is then scanned across the image to obtain a map of the time-dependent singlet exciton density as a function of position, convolved with the point spread function (PSF) of the imaging optics (see Methods). As fusion is a nonlinear process that requires the collision of two triplet excitons ( Supplementary Fig. 1 ), the triplet exciton density n T ( x , t ) is calculated from the measured singlet exciton density n S ( x , t ) using (see discussion below) [26] , [27] . 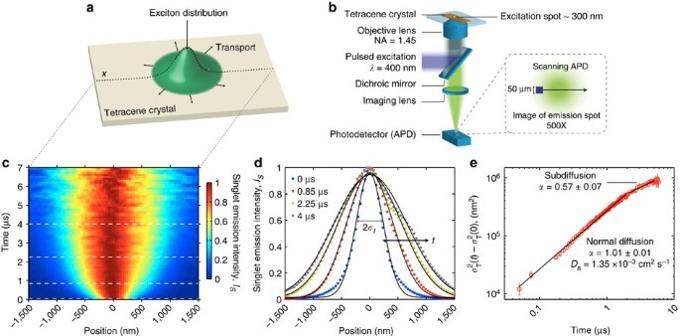Figure 2: Imaging tetracene exciton transport in time and space. (a) Conceptual schematic of the exciton transport measurement, showing the initial exciton distribution spreading in the plane of the crystal. (b) Schematic of the exciton diffusion imaging setup. The time-resolved APD is scanned across the emission spot to obtain a map of emission intensity as a function of position and time. (c) Map of emission intensity as it evolves in space and time as measured along the crystalaaxis. The distribution at a particular time has been normalized to emphasize changes in the distribution width. (d) Cross-sections of the emission intensity map at four time points showing spatial broadening of the intensity distribution.σIis the standard deviation of the Gaussian distribution. (e) Time evolution of mean square displacement of triplet excitons showing transition from normal to subdiffusive transport. Error bars reflect the 95% confidence interval of a Gaussian fit to the spatial intensity distribution. Figure 2: Imaging tetracene exciton transport in time and space. ( a ) Conceptual schematic of the exciton transport measurement, showing the initial exciton distribution spreading in the plane of the crystal. ( b ) Schematic of the exciton diffusion imaging setup. The time-resolved APD is scanned across the emission spot to obtain a map of emission intensity as a function of position and time. ( c ) Map of emission intensity as it evolves in space and time as measured along the crystal a axis. The distribution at a particular time has been normalized to emphasize changes in the distribution width. ( d ) Cross-sections of the emission intensity map at four time points showing spatial broadening of the intensity distribution. σ I is the standard deviation of the Gaussian distribution. ( e ) Time evolution of mean square displacement of triplet excitons showing transition from normal to subdiffusive transport. Error bars reflect the 95% confidence interval of a Gaussian fit to the spatial intensity distribution. Full size image Imaging transport in tetracene single crystal Figure 2c shows the spatial and temporal evolution of the emission intensity distribution, I ( x , t ), along the a axis of a tetracene single crystal after pulsed excitation at t =0. The spatial intensity distribution at each point in time has been normalized to a constant maximum value to emphasize changes in the width of the distribution. The initial near-Gaussian intensity distribution has a standard deviation of σ I ( t =0)=229 nm which rapidly broadens in the first 2 μs, with a subsequent slowing down of the expansion, reaching σ I ( t =7 μs)=701 nm ( Fig. 2d ). The broadening of the emission distribution is found to be independent of the excitation energy and hence cannot be attributed to nonlinear effects such as singlet–singlet exciton annihilation ( Supplementary Fig. 2 ). An alternative way to visualize the emission broadening is to plot the time-resolved emission in three spatial regions relative to the centre of the excitation spot ( Supplementary Fig. 3 ). This approach shows a buildup of intensity away from the excitation centre. We will now discuss how the singlet and triplet exciton density is extracted from the measured intensity distribution. The dynamics of the exciton distribution will then be discussed in the context of diffusion. Extracting the singlet distribution The measured image of emitted photons is a spatial convolution of the underlying singlet exciton distribution n s ( x , t ), the PSF of the emitted photons f PSF ( x ), and the APD detector f d ( x ): The PSF of emitted photons is an Airy disk pattern but can be approximated by a Gaussian function. The APD detector size is 50 μm × 50 μm, and when imaged in the sample plane at × 500 demagnification, the detected region originates from a sample area of 100 nm × 100 nm, which is small compared with the spot size, and hence can be neglected. Using the fact that the variance of convoluted Gaussians is additive, we find that where is the variance of the intensity distribution, is the variance of the singlet exciton distribution, and is the variance of the detection PSF. We can make the assumption that the width of the PSF is constant with time despite a small (~7 nm) dynamic red shift in the emission wavelength ( Supplementary Note 1 ). It then follows that the singlet exciton distribution variance can be obtained directly from the measured intensity distribution variance Importantly, we can see that does not depend on the width of the initial distribution. The convolution with the Gaussian PSF can also be neglected as long as the effect of exciton transport is larger than the broadening of the PSF due to red shifting of the emission. Extracting triplet density from singlet density The measured fluorescence intensity distribution is proportional to the singlet density in the material. However, energy transport in tetracene is dominated by triplet excitons. Hence we must determine the triplet exciton density on the basis of the singlet exciton density. We start by considering the simplified rate equation for the density of singlet excitons n S [26] : Here k S is the total singlet exciton decay rate, γ TTF is the triplet–triplet fusion rate constant, and n T is the triplet exciton density. As discussed by Burdett et al. [26] , the total singlet decay rate k S is dominated by the fission rate with k fiss ≈1/250 ps ( Fig. 1b ). We can make the assumption that because the measured delayed fluorescence lifetime is much longer than the fission lifetime for all times after the prompt fluorescence. Therefore the triplet density is given by: and the change in the triplet distribution variance is then The rate equation from which Equation (5) is derived is simplified and did not include the effect of exciton traps. In the presence of traps, the relationship between singlet exciton density and the free triplet exciton density (those not in a trap) becomes more linear as traps are filled. Therefore Equation (4) is modified at longer times [26] . However, generation of a singlet still requires the fusion two triplets, regardless of whether one of them is trapped. Therefore at a particular time, the variance of the total triplet exciton distribution (both free and trapped) is still given by Equation (6). In the above discussion we have ignored geminate recombination of correlated triplet pairs. As has been shown by Burdett et al. [28] , correlations between pairs of triplets can persist up to ~10 ns after fission. Such correlations modify the rate equation at early times and give a linear relationship between triplet and singlet exciton density. However, our measurements are primarily concerned with much longer time scales (~μs), and hence geminate recombination can be ignored in calculating the triplet density. Diffusion as the transport mechanism The observed exciton transport can be understood in the context of diffusion. The solution to the diffusion equation with a Gaussian initial condition is given by ( Supplementary Note 2 ) [29] where α is the diffusion exponent and D is a scaling factor. For normal diffusion, α =1 because the particle hopping rate is independent of time, and D is the diffusivity, expressed in units of cm 2 s −1 . In contrast, anomalous diffusion is characterized by α ≠1 and a time-dependent diffusivity. Subdiffusive transport ( α <1) is often caused by a disordered landscape through which the particles diffuse, resulting in trapping and decreased hopping rates with time. Superdiffusive transport such as ballistic motion is characterized by α >1. Figure 2e shows how the triplet exciton mean square displacement evolves in time in a tetracene crystal along the a axis. For t <2 μs after excitation, the triplet exciton transport follows a normal diffusive process with α =1.01±0.01 and a time-independent diffusion constant of D a =1.35±0.01 × 10 −3 cm 2 s −1 . Given the decay of the delayed fluorescence, the average distance for exciton diffusion along the a axis within the lifetime of the triplet excitons τ T =1.37 μs ( Fig. 1c ) is . While the diffusion constant of tetracene is an intrinsic property that depends on wavefunction overlap of adjacent molecules, the triplet lifetime can be limited by nonradiative recombination at trap sites and defects. In ultra-pure tetracene crystals the lifetime has been found to be up to 58 μs, which provides an upper limit to the a axis triplet diffusion in tetracene of 4.0 μm. Similar macroscopic exciton diffusion lengths have been measured in rubrene [16] , [19] . At longer times t >2 μs, we find that α=0.57±0.07, indicating a transition to a subdiffusive regime. Such anomalous diffusion is characteristic of particles diffusing in a disordered potential and is observed in a wide range of physical systems from protein diffusion in cells to charge diffusion in semiconductors [30] , but to our knowledge has not previously been observed in excitonic systems. Recent theoretical work has predicted that subdiffusive transport of excitons can occur in energy disordered systems with excitonic energy trap levels at the low energy tail of the exciton distribution [31] . In tetracene we attribute the subdiffusive transport to the excitons becoming trapped in lower-energy molecular sites, which decreases the hopping rate for a subpopulation of excitons. We show below that this picture of subdiffusion is consistent with our measurements of spectral distribution of excitons (see below). Anisotropy in exciton diffusion Due to the herringbone arrangement of molecules in tetracene, the π-orbital overlap is greater in the ab plane compared to the c axis ( Fig. 3 ). Consequently, a large anisotropy for Dexter transfer rate and hence diffusivity is predicted [9] , but until now has only been observed experimentally in steady-state measurements of rubrene single crystals [19] . Our measurements show exciton diffusion in both space and time along the b axis and the c axis ( Fig. 3 ). The exciton transport along both axes follows normal diffusion with α ≈1, but with a seven-fold anisotropy between the b axis, D b =2.28±0.07 × 10 −3 cm 2 s −1 , and the c axis, D c =0.31±0.02 × 10 −3 cm 2 s −1 . The trend in diffusivity between the three axes follows the theoretical predictions of Yost et al. [9] Previous measurements of exciton transport along the c axis in tetracene have shown wide variation. These results, along with comparison to our results and theory, are summarized in Supplementary Table 1 . 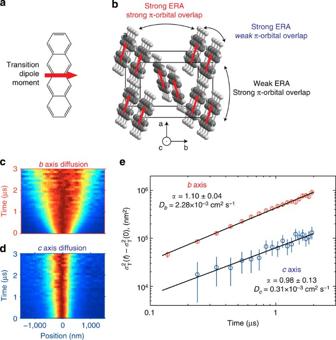Figure 3: Anisotropy in diffusion. (a) Structure of tetracene monomer and the orientation of the transition dipole moment. (b) Crystal structure of tetracene showing the three crystallographic axes. The red arrow represents the optical transition dipole moment. The largest π-orbital overlap occurs along theaandbaxes, resulting in large anisotropy in Dexter transfer between theabplane and thecaxis. The strongest ERA would occur along thebandcaxes due to alignment of the dipoles, while the strongest wavefunction overlap is along theaandbaxes. (c,d) Normalized spacio-temporal maps of emission intensity as measured along thebaxis (c) andcaxis (d). (e) Time evolution of the triplet exciton mean squared displacement along thebandcaxes, showing large anisotropy. Error bars reflect the 95% confidence interval of a Gaussian fit to the spatial intensity distribution. Figure 3: Anisotropy in diffusion. ( a ) Structure of tetracene monomer and the orientation of the transition dipole moment. ( b ) Crystal structure of tetracene showing the three crystallographic axes. The red arrow represents the optical transition dipole moment. The largest π-orbital overlap occurs along the a and b axes, resulting in large anisotropy in Dexter transfer between the ab plane and the c axis. The strongest ERA would occur along the b and c axes due to alignment of the dipoles, while the strongest wavefunction overlap is along the a and b axes. ( c , d ) Normalized spacio-temporal maps of emission intensity as measured along the b axis ( c ) and c axis ( d ). ( e ) Time evolution of the triplet exciton mean squared displacement along the b and c axes, showing large anisotropy. Error bars reflect the 95% confidence interval of a Gaussian fit to the spatial intensity distribution. Full size image Role of radiative energy transfer Along with near-field hopping, the emission and reabsorption of a photon is another mechanism that can give rise to energy transport. This radiative form of energy transport is often difficult to distinguish from exciton hopping in exciton transport measurements, as has been discussed by Powell et al. [32] In particular, photon emission followed by reabsorption (ERA) is itself a random walk process due to the randomization of the photon direction with each emission event. In materials dominated by singlet excitons, hopping transport and ERA transport occurs along the same axes because both mechanisms rely on the interaction of two dipoles—hopping in the near-field and ERA in the far-field. Tetracene, in contrast, is dominated by triplet excitons, the transport of which depends on wavefunction overlap. Transition dipole alignment and wavefunction overlap do not necessarily occur most efficiently along the same axes. Unlike most conjugated organic molecules, the dipole moment of tetracene is perpendicular to the long molecular axis. On the basis of the orientation of the dipole moment and the crystal structure we can see from Fig. 3b that the strongest dipole alignment, and hence ERA rate, occurs along the b crystal axis and the c crystal axis, with the weakest ERA occurring along the a axis. Consequently, the largest anisotropy in ERA is expected to be between the a and b axes, and a much smaller anisotropy is expected between the b and c axes. Indeed, the observed anisotropy in both absorption and emission between the a and b axes is ~3-fold as measured by Tavazzi et al. [33] In contrast, the largest π-orbital overlap anisotropy and hence the triplet exciton hopping anisotropy is between the b and c axes ( Fig. 3b ). On the basis of the observed anisotropy, we can conclude that most of the observed distribution broadening is due to triplet exciton hopping and not ERA. However, small contributions to the observed energy transport from radiative transfer cannot be ruled out, and hence the measured diffusivities give an upper bound on the diffusivity due to Dexter transfer. Spectral dynamics during transport In addition to spatial broadening of the exciton distribution, we find that the spectrum of the delayed fluorescence also evolves in time and space. 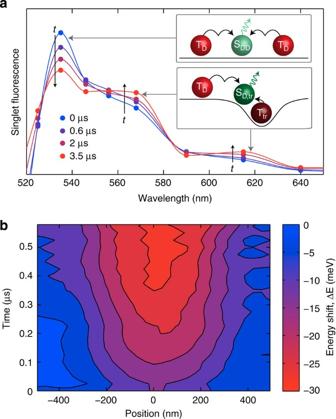Figure 4: Filling of exciton traps as diffusion proceeds. (a) Tetracene crystal emission spectrum at four time points after excitation, integrated over all space. Circles are measured values and lines are spline interpolates. Schematic represents two processes that form singlets. The emission peak atλ=535 nm is assigned to high energy singlets SDDwhich are formed by the fusion of two freely diffusing triplets TD. The emission peaks atλ=570 nm andλ=615 nm are assigned to lower-energy singlets SD,trwhich are formed by the fusion of a long-lived trapped triplet Ttrand a freely diffusing triplet TD. (b), Spatio-temporal map of the average energy of the emission spectrum showing more rapid red shifting in the centre of the distribution. The relative luminescence intensities of the three vibronic peaks atλ=535 nm,λ=570 nm andλ=615 nm favour the red-shifted emission at later times. This is consistent with the schematic ina, which shows that the higher-energy fluorescence is the result of fusion of two diffusing triplet excitons, whereas the lower-energy fluorescence is due to the fusion of a diffusing triplet exciton and a trapped triplet exciton. Figure 4a shows that the fluorescence spectrum at t =0 has a single peak at λ =535 nm which decays with a concomitant increase of lower-energy vibronic peaks at λ =570 nm and λ =615 nm. To understand the origin of the low energy emission, we visualize the spectral evolution by measuring the shift of the average energy of the emission spectrum at each position and time. Figure 4b shows that as exciton diffusion proceeds, the emission spectrum red shifts faster near the centre of the spatial distribution ( x =0) than in regions on the periphery of the distribution. This observation is consistent with the presence of exciton energy traps [34] . Namely, as the diffusion proceeds, exciton traps are filled faster in the centre of the distribution, where the triplet density is higher and more trap sites can be sampled. These long-lived trapped excitons undergo fusion with freely diffusing excitons, resulting in lower-energy singlet excitons. This picture is also consistent with our finding that the emission from red-shifted regions has a more linear scaling with increasing triplet exciton density (adjusted by increasing the excitation light intensity), confirming that the low energy emission is due to the fusion of diffusing triplets and a fixed number of trapped excitons ( Supplementary Fig. 4 ). Such low energy emission has also been identified in rubrene, and in that work it is similarly attributed to the presence of structural defects that act as exciton traps [35] . Figure 4: Filling of exciton traps as diffusion proceeds. ( a ) Tetracene crystal emission spectrum at four time points after excitation, integrated over all space. Circles are measured values and lines are spline interpolates. Schematic represents two processes that form singlets. The emission peak at λ =535 nm is assigned to high energy singlets S DD which are formed by the fusion of two freely diffusing triplets T D . The emission peaks at λ =570 nm and λ =615 nm are assigned to lower-energy singlets S D,tr which are formed by the fusion of a long-lived trapped triplet T tr and a freely diffusing triplet T D . ( b ), Spatio-temporal map of the average energy of the emission spectrum showing more rapid red shifting in the centre of the distribution. The relative luminescence intensities of the three vibronic peaks at λ =535 nm, λ =570 nm and λ =615 nm favour the red-shifted emission at later times. This is consistent with the schematic in a , which shows that the higher-energy fluorescence is the result of fusion of two diffusing triplet excitons, whereas the lower-energy fluorescence is due to the fusion of a diffusing triplet exciton and a trapped triplet exciton. Full size image Transport under increasing disorder One of the defining features of organic and nanocrystalline materials is their high morphological and energetic disorder. Consequently understanding how exciton transport is affected by disorder is crucial for the design of new excitonic materials. To this end we measure how exciton diffusion is affected as the disorder in tetracene is increased relative to the single crystal ( Fig. 5a,b and Supplementary Fig. 5 ). 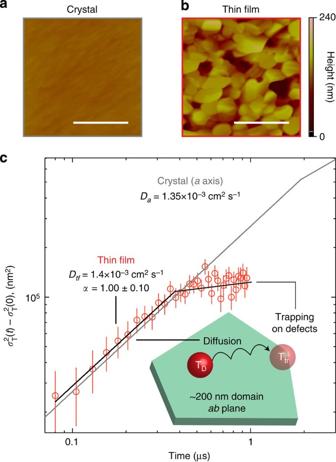Figure 5: Diffusion in tetracene polycrystalline film. (a,b) Atomic force microscopy images of (a) a single crystalabplane and (b) of a tetracene evaporated film (500 nm average thickness). Scale bars, 1 μm. Crystalline domains in the film are ~200 nm in size. (c) Time evolution of the triplet exciton mean squared displacement for the film and comparison to the fit of the crystalaaxis data (grey line), showing an earlier transition to subdiffusion for the thin film relative to the crystal. Error bars reflect the 95% confidence interval of a Gaussian fit to the spatial intensity distribution. Schematic shows a tetracene thin film crystalline domain in which a freely diffusion exciton TDreaches a domain wall or bulk defect and becomes a trapped exciton Ttr. Figure 5c shows how the mean squared displacement of the exciton distribution evolves in time for a thermally evaporated film of tetracene that is polycrystalline. By atomic force microscopy the crystalline domain size is measured to be ~200 nm ( Fig. 5b ), small compared with the a axis diffusion length of L a =610 nm, measured above. We find that transport in the thin film sample proceeds by normal diffusion for t <350 ns with a diffusivity D tf =1.4 × 10 −3 cm 2 s −1 . This value falls between the diffusivities found for the a and b crystal axes, consistent with our X-ray diffraction measurements showing that the film is composed of randomly oriented crystalline domains in the ab plane. This agreement in diffusivities indicates that the trap density within the bulk of a single domain of the film is similar to that of single crystal. However, in contrast to the single crystal, transport in the film transitions to subdiffusive at t ~350 ns, much earlier than the transition for the single crystal at t ~2 μs, as observed in Fig. 2e . The average diffusion distance of excitons in t =350 ns is 440 nm, which indicates that a large fraction of diffusing excitons have encountered a domain wall or other defects in the crystallite on which they were formed. Due to the discontinuity in crystal order at the domain wall, excitons can become trapped at the domain boundary [26] or confined by the domain boundary [36] , leading to exciton trapping and the subsequent observation of subdiffusion. Figure 5: Diffusion in tetracene polycrystalline film. ( a , b ) Atomic force microscopy images of ( a ) a single crystal ab plane and ( b ) of a tetracene evaporated film (500 nm average thickness). Scale bars, 1 μm. Crystalline domains in the film are ~200 nm in size. ( c ) Time evolution of the triplet exciton mean squared displacement for the film and comparison to the fit of the crystal a axis data (grey line), showing an earlier transition to subdiffusion for the thin film relative to the crystal. Error bars reflect the 95% confidence interval of a Gaussian fit to the spatial intensity distribution. Schematic shows a tetracene thin film crystalline domain in which a freely diffusion exciton T D reaches a domain wall or bulk defect and becomes a trapped exciton T tr . Full size image In conclusion, our measurements demonstrate that transport of triplet excitons in tetracene occurs by normal diffusion with a transition to subdiffusive transport that depends on sample morphology and, consequently, trap density. These results are the first direct spatial, temporal and spectral observation of exciton transport in a molecular system, which can be taken as an archetype for both natural and engineered, ordered and disordered systems that rely on exciton transport. In addition, the imaging technique developed for this study is a general tool that can be applied to exciton transport in a wide range of materials, including those dominated by singlet exciton diffusion, characterized by much shorter exciton diffusion lengths of 10 to 50 nm [4] . As only the change in exciton distribution width must be determined, no fundamental limit exists on the shortest diffusion length that can be measured with this technique. Sample preparation Tetracene was purchased from Luminescence Technology Corporation and further purified three times by vacuum physical vapour transport [37] . Thin film samples were fabricated on 170 μm thick microscope cover glass with no additional cleaning. The tetracene thin films were grown by thermal evaporation in a vacuum chamber with a deposition pressure of less than 3 × 10 −6 Torr at a rate between 2 and 4 Å s −1 . The film thickness was determined in-situ through use of a quartz crystal oscillator. The substrate holder was rotated during thermal evaporation resulting in a film thickness variation of ±10% across the width of the substrate holder [24] . The thermal evaporator was directly attached to a nitrogen-filled glovebox (with less than 1 p.p.m. O 2 and H 2 O, where the tetracene films were packaged in the dry nitrogen environment using ultraviolet (UV) curing epoxy and a glass cover slip. The thin film was shadowed from the UV light during epoxy exposure by shadowing it with a square of aluminium foil. Single crystals of tetracene are grown using the same purified tetracene by the vapour phase method in an Ar environment [37] . The resulting crystallites had one large facet with a typical size of 1 × 1 mm 2 and a thickness of 20 μm. To avoid fluorescence waveguiding due to an air gap between the crystallite and the cover glass, the cover glass is first wetted with immersion oil (Nikon, with a refractive index of n =1.52). The crystallites are then placed in the oil and pressed with another cover glass to make a sealed sample. We find that the tetracene was completely insoluble in the immersion oil and that the oil had no effect on the fluorescence spectrum or intensity. Most optical measurements of organic crystals are performed in the plane perpendicular to the growth direction because of the difficulty in handling and orienting a thin crystallite. Here we are interested in observing the large predicted anisotropy in diffusion between the c axis and the ab plane. To image diffusion along the crystal c axis, a crystallite was wedged between two pieces of glass and then immersed in the objective oil ( Supplementary Fig. 6 ). From the small anisotropy in fluorescence polarization in the image plane it was determined that the orthogonal axis to the c axis for this crystal was the b axis. Determination of crystal axes To determine the crystallographic axes of the single crystals and thin films, a combination of X-ray diffraction and polarized light microscopy was used. X-ray diffraction patterns were taken of the single crystal and thin film tetracene on glass cover slides in air ( Supplementary Fig. 7 ). The crystal was oriented so that the largest facet was in contact with the substrate. The X-ray source was copper k-alpha radiation and the scan was measured in a coupled theta-two geometry. The (001) diffraction peak and its higher orders were the only visible diffraction peaks. Scans measured to 60° 2θ found no additional diffraction. Thus we conclude that both the 500 nm film and the crystal have the crystal c axis oriented perpendicular to the substrate. To determine the orientation of the in-plane axes, the samples are imaged using the same inverted microscope and 100X oil immersion objective as used for diffusion imaging ( Supplementary Figs 8 and 9 ). The samples were excited with a mercury lamp at a wavelength of 470±15 nm and fluorescence was collected at all wavelengths above 500 nm. The fluorescence is imaged onto a CCD camera. A thin film linear polarizer is placed between the objective lens and the camera to image selected polarization of fluorescence. Diffusion imaging setup Exciton transport in tetracene thin films and crystals was measured using a custom-built fluorescence microscope ( Supplementary Fig. 10 ). The setup is similar to a laser scanning confocal microscope but with a key modification. The ~500 nm full width at half maximum (FWHM) fluorescence spot is magnified 500-fold using the objective lens and a lens external to the microscope to produce a spot with an FWHM of ~250 μm. A time-resolved photodetector with a square active area of 50 μm × 50 μm is then scanned across the magnified fluorescence spot to obtain a map of fluorescence intensity as a function of time and position on the sample. The fluorescence intensity map is then assigned to a density of excitons, depending on whether singlet or triplet excitons are the primary species in the material. The laser excitation source is a Ti:Sapphire laser producing pulses ~100 fs in duration at a repetition rate of 80 MHz at a wavelength of λ =800 nm. To observe the long (~μs) dynamics of tetracene emission, the high repetition rate pulses are passed through an electro-optic pulse picker (Conoptics Model 350–160 KDP Series Electro-Optic Modulator, with driver Model 25D, and Model 305 Synchronous Countdown System). Typical repetition rates used for measurements of tetracene diffusion are 114 kHz, corresponding to a delay between pulses of 8.8 μs. The reduced repetition rate pulses are focused with an f =100 mm lens onto a frequency doubling BBO crystal (Crystech Inc.) resulting in λ =400 nm light. The crystal is cut for collinear phase-matching between the incoming and outgoing upconverted light. The λ =400 nm beam is collimated and passed through a 750 nm shortpass filter to remove the residual λ =800 nm laser light and then passed through a λ =390±20 nm bandpass filter (Semrock, Inc. FF01-390/40-25). The beam is then sent into an f =18.4 mm fibre coupler (Thorlabs Inc. PAF-X-18-PC-A) to couple into a single mode fibre with a length of 20 cm. The output of the single mode fibre is collimated with a diffraction limited compound collimator to a diameter of 10 mm. The single mode beam is directed into the back of an inverted optical microscope (Nikon Ti-E) and reflected into the objective lens by a longpass dichroic mirror with a cutoff wavelength of λ =415 nm (Semrock Inc., Di02-R405-25 × 36). The 100X oil immersion objective lens (Nikon CFI PlanApo Lambda 100X Oil, numerical aperture (NA)=1.45, effective focal length f =2 mm) focuses the laser beam to a near-diffraction-limited spot with a FWHM of 200 nm, as determined from imaging the reflection spot ( Supplementary Fig. 11 ). The sample is mounted above the objective lens on a piezoelectric scanning stage. Each measurement of tetracene crystals and thin films was done on a single spot and the piezoelectric stage was used only to move to new areas between measurements. The fluorescence from the sample is collected by the same objective and the resulting collimated beam passes through the dichroic mirror and then through a longpass filter with a cutoff at λ =416 nm (Semrock Inc., BLP01-405R-25) to remove any residual scattered or reflected excitation light. The fluorescence beam is then focused by an achromatic lens with a focal length f =1,000 mm to a region outside the microscope. The focal plane of the f =1,000 mm lens is determined by scanning an imaging CCD along the optical axis to find the smallest fluorescence spot size. A single photon detecting avalanche photodiode (APD) (MPD PDM Series 50 μm) is mounted in the focal plane on a two-dimensional computer-controlled translation stage. The output of the APD is connected to a timing module with a resolution of 4 ps (PicoQuant PicoHarp 300), which detects the arrival time of each photon. This technique, known as time-correlated single photon counting results in a histogram of photon arrival times which corresponds to the time-dependent rate of photon emission from the sample. The trigger for the timing module is created by splitting part of the λ =800 nm laser beam before the BBO crystal onto a PIN photodiode (Hamamatsu C1808-03), which generates power independent electrical trigger pulses with a jitter of <5 ps. The overall timing resolution of the system is ~30 ps, as determined by measuring scattered laser light. The APD detector is scanned with a velocity of 2.5 μm s −1 across the excitation spot in either the vertical or horizontal direction. The time-resolved fluorescence trace is recorded at each detector position resulting in a map of fluorescence intensity along one axis of the sample as a function of time. The detector is shielded from stray light, resulting in a dark count rate in the presence of the excitation laser of ~100 counts per second. The spatial resolution of the imaging setup was determined by imaging the photoluminescence from single colloidal CdSe quantum dots, which are less than 10 nm in diameter, immobilized on a glass substrate. The resolution is near-diffraction limited with a FWHM of the PSF of γ =250 nm. This value agrees well with the theoretical Rayleigh resolution of 0.61 λ /NA=265 nm, when using an NA=1.4 objective. All measurements are done with an incident average power on the sample of 1 nW, corresponding to a pulse energy of 9 fJ. On the basis of the absorption coefficient at λ =400 nm α 400 nm =7.5 × 10 3 cm −1 the estimated singlet exciton density at t =0 is then n (0)=1.5 × 10 17 cm −3 . This density is well below the tetracene molecular density of ~10 21 cm −3 , and well below the onset of exciton–exciton annihilation effects. Samples had excellent photostability under this excitation power and consequently each measurement (~30 min in duration) was done on the same ~300 nm diameter spot on the sample. How to cite this article: Akselrod, G. M. et al. Visualization of exciton transport in ordered and disordered molecular solids. Nat. Commun. 5:3646 doi: 10.1038/ncomms4646 (2014).